Silver hake tracks changes in Northwest Atlantic circulation Recent studies documenting shifts in spatial distribution of many organisms in response to a warming climate highlight the need to understand the mechanisms underlying species distribution at large spatial scales. Here we present one noteworthy example of remote oceanographic processes governing the spatial distribution of adult silver hake, Merluccius bilinearis , a commercially important fish in the Northeast US shelf region. Changes in spatial distribution of silver hake over the last 40 years are highly correlated with the position of the Gulf Stream. These changes in distribution are in direct response to local changes in bottom temperature on the continental shelf that are responding to the same large scale circulation change affecting the Gulf Stream path, namely changes in the Atlantic meridional overturning circulation (AMOC). If the AMOC weakens, as is suggested by global climate models, silver hake distribution will remain in a poleward position, the extent to which could be forecast at both decadal and multidecadal scales. Many recent studies [1] , [2] , [3] , [4] , [5] , [6] have documented shifts in spatial distribution of marine organisms in response to changing temperatures. One study [1] documented poleward shifts in spatial distribution of many Northeast US fish populations over the last forty years that were concurrent with the recent warm phase of the Atlantic multi-decadal oscillation (AMO). The AMO is an index based on sea surface temperature averaged over the entire North Atlantic (0–60°N) [7] , but it is thought to be linked to the variability in the basin-wide ocean circulation, that is, Atlantic meridional overturning circulation (AMOC) [8] . AMOC variability is suggested to be transmitted to the Northeast US shelf region through temperature and flow variations arising from the Labrador Sea and Subpolar gyre to the north [9] . Variability in the vicinity of the Gulf Stream (GS) is dominated by the changes in the north-south position of the GS on interannual to decadal time scales, whereas the changes in velocity, volume transport, and width of the GS are relatively small [10] . The north-south GS position change is strongly correlated with changes in sea surface temperature and circulation in the Slope water region between the GS and the shelf [11] , but the influence of the GS on the continental shelf ecosystem is not well understood. An index for the GS position extending back to the mid-1950s has been constructed on the basis of historical subsurface temperature data at 200 m depth and used to understand several observed variations in physical climate [9] , [11] , [12] , [13] . The GS is known to be an important feature for marine species especially passive marine organisms such as plankton [14] , [15] including fish larvae [16] . We examined the correlation of the GS position with one species, the silver hake, a semi-pelagic fish in which a poleward shift in both the northern and southern populations has already been observed [1] . We also investigated the relationship between the GS path changes, temperature on the shelf and silver hake spatial distribution to understand the likely mechanistic link between the GS position and silver hake distribution. Our findings indicate that silver hake respond to remote oceanographic processes by shifting their spatial distribution to remain within their preferred temperature range. Shift in silver hake spatial distribution Similar shifts in distribution of silver hake were observed in both the spring and fall, but maps of its spring distribution representing the past and current time periods illustrate the shift in biomass well ( Fig. 1 ). Where there were once high densities of silver hake in the southern extent of the Northeast Fisheries Science Center (NEFSC) bottom trawl survey in the early period of 1968–1972, in the later period of 2003–2008, there were very few silver hake. Over the same time period, the maximum concentration of silver hake shifted into the northern part of the Northeast US, namely the Gulf of Maine. Centre of mass (COM) and biomass (mean-stratified weight per tow) were calculated for the northern and southern populations of silver hake as described by Nye et al . [1] The COM changed very little over time for the northern silver hake, but there has been a gradual increase in the COM for southern silver hake indicative of its poleward shift in distribution ( Fig. 2 ). On top of the long-term increase over the last 40 years, fluctuations on a decadal time scale are also apparent. For instance, southern silver hake COM was furthest north ( Fig. 2a ) and northern silver hake biomass was highest ( Fig. 2d ) in 1998–2002, while both decreased in the last ∼ 5 years. 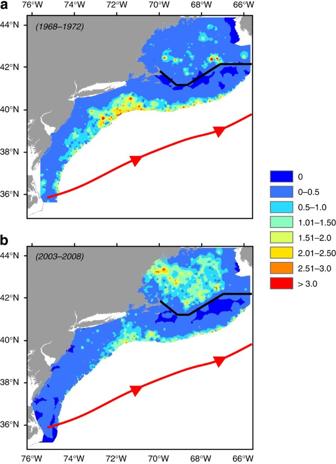Figure 1: Changing spatial distribution of silver hake. (a) Past (1968–1972) and (b) recent (2003–08) spatial distribution of silver hake biomass in the spring (March–May). Contoured colours represent the log weight (kg) per tow. Note the poleward shift in biomass. Inverse distance weighting was used to smooth the biomass of silver hake. The black line demarcates the boundary between the northern and southern populations of silver hake. The red line indicates the mean position of the Gulf Stream. Figure 1: Changing spatial distribution of silver hake. ( a ) Past (1968–1972) and ( b ) recent (2003–08) spatial distribution of silver hake biomass in the spring (March–May). Contoured colours represent the log weight (kg) per tow. Note the poleward shift in biomass. Inverse distance weighting was used to smooth the biomass of silver hake. The black line demarcates the boundary between the northern and southern populations of silver hake. The red line indicates the mean position of the Gulf Stream. 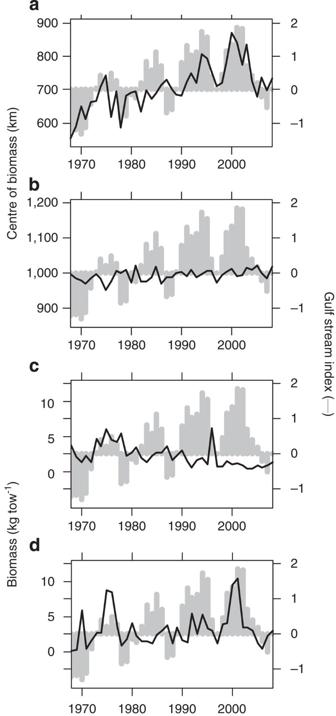Figure 2: Relationship of GS position with silver hake biomass and spatial distribution. Relationship of the meridional position of the north wall of the GS in spring (grey bars) with measures of spring silver hake spatial distribution and abundance including the (a) COM for the southern population, (b) COM of the northern population, (c) BM of the southern population and (d) BM of the northern population of silver hake. Full size image Figure 2: Relationship of GS position with silver hake biomass and spatial distribution. Relationship of the meridional position of the north wall of the GS in spring (grey bars) with measures of spring silver hake spatial distribution and abundance including the ( a ) COM for the southern population, ( b ) COM of the northern population, ( c ) BM of the southern population and ( d ) BM of the northern population of silver hake. Full size image Relationship between hake distribution and Gulf Stream position The north-south position of the GS displays a similar trend and interannual-decadal variability as the COM of the southern population of silver hake on the shelf ( Fig. 2a ). Cross correlation analysis on the 41-year time series revealed that the GS index is significantly correlated with southern silver hake COM ( r max =0.72, P <0.001) and the biomass of northern silver hake ( r max =0.43, P =0.005, Fig. 2d ). When the time series were linearly detrended, the GS position was still significantly correlated with the COM for southern silver hake ( r max =0.60, P <0.001) and biomass of the northern silver hake population ( r max =0.44, P =0.0062). When the spring GS index was correlated with the spring silver hake data, the maximum correlation occurred at lag=0, but when the fall GS values were correlated with spring silver hake data, the peak correlation occurred when the GS led silver hake COM and biomass by 1 year, both with and without detrending. This implies that the GS leads silver hake distribution by 6 months. Furthermore, the fact that the correlation remained strong after detrending in both the spring and fall analyses suggests that the decadal variability may be predictable. Relationship between shelf temperatures and Gulf Stream position Adult silver hake shift their spatial distribution seasonally [17] , and it has been assumed that seasonal movements occur in response to seasonal changes in water temperature, because silver hake are rarely found in waters less than 4 °C, with their temperature preference being 7–10 °C [18] , [19] , [20] . Thus, we hypothesized that the GS path changes are reflected in silver hake spatial distribution not by physical transport of the early life stages, but through its relationship to change in bottom-water temperature to which adult fish respond. Indeed, the position of the GS was highly correlated with mean-stratified bottom temperature averaged over the entire shelf ( r max =0.51, lag=0, P <0.001). We relate the GS path directly to silver hake habitat by examining the average temperature for stations >100 m in the southern region versus the northern region of the survey. Bottom temperature averaged within the southern population boundary, the area from which silver hake moved, increased from about 10 °C when the GS was in a more southerly position, to more than 12 °C when the GS was more northerly, well above the preferred temperature range of silver hake, ( Fig. 3a ). Average temperatures within the northern population area also increased with the GS index, but approached the preferred temperature range of silver hake ( Fig. 3a ). Spatiotemporal changes in temperature are also illustrated in Nye et al . [1] Even though shelf temperatures have changed, the average temperature at which the southern silver hake population was found (or catch temperature) remained within the 6–10 °C temperature range and there appears to be no relationship of catch temperature with the GS ( Fig. 3a ). However, silver hake COM has changed proportional to the GS position changes ( Fig. 3b ), indicating that silver hake remain within their preferred temperature range by shifting their distribution. The proportion of silver hake biomass found in the northern population boundaries increased as the GS shifted north, suggesting that the southern population may move into the northern population boundary ( Fig. 3c ). 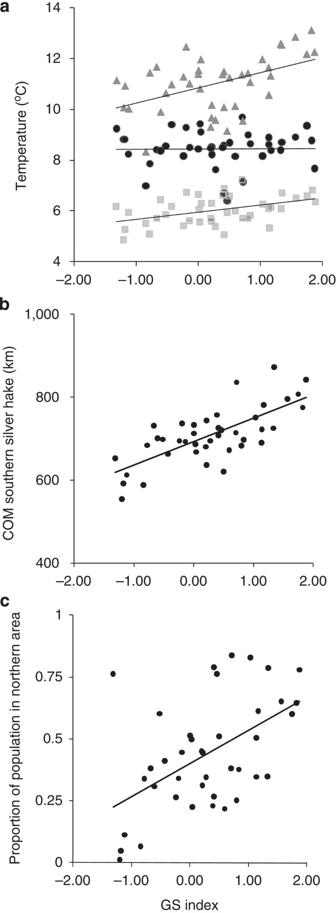Figure 3: Linking GS position with local bottom water temperature and silver hake thermal habitat. The relationship between the Gulf Stream index and the (a) bottom temperature (only stations >100 m) in the southern region (grey triangles) and northern region (grey squares) is shown along with the catch temperature of southern silver hake (black points). Temperature in both the northern and southern regions increase with GS index with temperatures in the southern region elevated above silver hake temperature preferences. In contrast, the average temperature at which silver hake were found remains the same indicating that, as temperatures increase in the south, silver hake shift their distribution poleward as indicated by (b) COM of southern silver hake. Northern silver hake biomass increases and southern silver hake biomass decreases as southern silver hake enter the northern population area as reflected in the (c) proportion of silver hake (southern and northern populations combined) in the northern population area. Figure 3: Linking GS position with local bottom water temperature and silver hake thermal habitat. The relationship between the Gulf Stream index and the ( a ) bottom temperature (only stations >100 m) in the southern region (grey triangles) and northern region (grey squares) is shown along with the catch temperature of southern silver hake (black points). Temperature in both the northern and southern regions increase with GS index with temperatures in the southern region elevated above silver hake temperature preferences. In contrast, the average temperature at which silver hake were found remains the same indicating that, as temperatures increase in the south, silver hake shift their distribution poleward as indicated by ( b ) COM of southern silver hake. Northern silver hake biomass increases and southern silver hake biomass decreases as southern silver hake enter the northern population area as reflected in the ( c ) proportion of silver hake (southern and northern populations combined) in the northern population area. Full size image Alternative mechanisms Two alternative mechanisms for the observed GS-silver hake correlation were also considered, but were eliminated as factors influencing silver hake spatial distribution. First, silver hake is a commercially important fish so the effects of fishing on biomass and spatial distribution must be considered. Changes in population size as a result of fishing pressure might explain changes in spatial distribution. Biomass of the southern silver hake population has declined since the beginning of the survey, but, biomass of the northern silver hake population has fluctuated greatly at a higher overall level of biomass ( Fig. 2b,d ). Landings data extend back to the 1950s and have been consistently higher in the southern area than the northern area since the 1960s ( Supplementary Fig. S1 ). However, landings data can fluctuate due to changes in fish availability, behaviour of fishermen, fishing technology and regulations. Therefore, the exploitation index (landings/survey biomass) is a better index of fishing pressure than landings, because it takes into account the biomass available to the fishery. A high exploitation index indicates high fishing pressure because removals by the fishery are large, relative to the biomass of fish available. We tested the hypothesis that higher fishing pressure in the southern population caused an apparent northward shift in distribution. The exploitation index in both populations peaked in the early 1960s and has declined since ∼ 1980 ( Supplementary Fig. S1 ). Higher exploitation rates in the southern regions would reduce population size and may give the appearance of the southern population shifting northward. This hypothesis would be supported if the exploitation index was positively correlated with the COM of southern silver hake after both time series were linearly detrended. The only statistically significant correlation between exploitation rate and COM of the southern population occurred when the exploitation index led COM by 1 year. However, this correlation was negative ( r max =−0.43, P =0.0028), not positive as would be expected, meaning that, as exploitation decreased, COM increased ( Fig. 4 ). Furthermore, a shift in distribution in response to high fishing would be expected much earlier in the time series as a result of extremely high exploitation rates in the 1960s even if the effect of fishing on distribution was lagged by several years. This hypothesis also does not explain the tight correlation between the COM and the position of the GS. 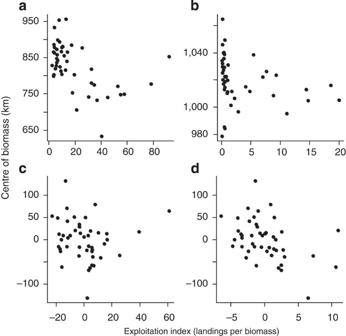Figure 4: The relationship between fishing pressure and silver hake distribution. The relationship of Exploitation index (Landings/survey biomass) with silver hake centre of mass (COM) for both the southern (a,c) and northern populations (b,d) of silver hake before (top two panels) and after linear detrending (bottom two panels). There is a weak negative correlation after detrending indicated that as fishing pressure decreased, silver hake distribution shifted northward. Figure 4: The relationship between fishing pressure and silver hake distribution. The relationship of Exploitation index (Landings/survey biomass) with silver hake centre of mass (COM) for both the southern ( a , c ) and northern populations ( b , d ) of silver hake before (top two panels) and after linear detrending (bottom two panels). There is a weak negative correlation after detrending indicated that as fishing pressure decreased, silver hake distribution shifted northward. Full size image We also tested the hypothesis that the apparent shift in distribution of the southern population and the increase in biomass (BM) of the northern population may simply be the result of higher population productivity in the northern population than in the southern population in response to GS. This explanation is plausible since the BM in the northern population is positively correlated and the BM of the southern population is weakly negatively correlated with the GS index. Higher population productivity would most likely be expressed in higher reproductive success or recruitment (R). If the GS affected spatial distribution by differential effects on reproductive success the survivor ratio (log (R/SSB+1)) should be negatively correlated in the southern population and positively correlated in the northern population with the GS. However, the GS was positively correlated with the survivor ratios for both the southern population ( r max =0.38, P =0.010) and the northern population ( r max =0.45, P =0.0023) with the maximum correlation occurring at lag=0 ( Fig. 5 ). As a further test of this hypothesis, recruitment should be negatively correlated to COM in the southern population and positively correlated with BM in the northern population, but there was no relationship between recruitment and either of these metrics. Therefore, the GS may positively influence recruitment of silver hake in general because both the northern and southern populations were similarly positively correlated with the GS. However, the shifts in distribution and the strong correlation between COM with the GS that we have described are not a result of differential population responses to this environmental forcing. 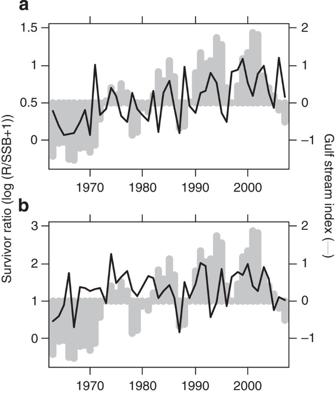Figure 5: Relationship between recruitment success and the Gulf Stream index. Recruitment was positively correlated with the position of the GS in both the (a) southern and (b) northern populations of silver hake, but the correlation was weak. The survivor ratio (log (R/SSB+1)) is used as a measure of recruitment. Figure 5: Relationship between recruitment success and the Gulf Stream index. Recruitment was positively correlated with the position of the GS in both the ( a ) southern and ( b ) northern populations of silver hake, but the correlation was weak. The survivor ratio (log (R/SSB+1)) is used as a measure of recruitment. Full size image In this study, we have used the GS path as a leading indicator of conditions at the shelf break, but in reality both silver hake and the GS are responding to processes 'upstream' from our study area arising in the Labrador Sea [21] and reflecting large-scale circulation changes associated with the AMOC. Note that the GS is located far off-shore from the study region ( Fig. 1 ), which minimizes direct GS influence on the shelf. Changes in the Slope-water temperatures north of our study area were found to account for 50% of the variance of temperature changes over the adjacent continental shelf with a lag of several months [22] . Long records (1875–2007) from lightships over the US continental shelf along the east coast indicate that substantial interannual variability of temperatures arises due to advection from the north [23] . When flow into the region from the Labrador Sea decreases, the northeast U.S. shelf is warmer, the GS is located closer to the shelf, and the preferred habitat of silver hake is shifted northwards. Conversely, when flow from the Labrador Sea increases, the northeast U.S. shelf is cooler, the GS is farther from the shelf, and the preferred habitat of silver hake is shifted southwards. Thus, there is a clear suggestion that climatic signals influence the bottom waters over the shelf and that silver hake are responding to this remote forcing. The GS location is the best leading indicator of conditions on the shelf because changes in the location of the GS can be continuously monitored and more easily quantified than changes in the flow of Labrador Current into the northeast U.S. shelf ecosystem. Global climate models predict that AMOC will likely weaken by about 25% until 2100 (ref. 24 ). Recently, Joyce and Zhang [9] showed that AMOC using the temperature at 400 m as a proxy is highly negatively correlated with the GS position. This suggests that in the future the GS will be in a more northerly position, and thus we infer that silver hake population will reside predominantly in the Gulf of Maine and be scarce in the southern regions of the Northeast US continental shelf. The implications of silver hake shifting their distribution poleward are numerous. First, silver hake supports a valuable commercial fishery. In 2007, landings exceeded 6,000 metric tons and $7 million [25] . However, approximately 75% of those landings occurred in the southern areas of the Northeast US shelf, not in the northern area, where we might expect silver hake to reside in the future. Second, this work presents a potential mechanism for substantial mixing between the northern and southern populations of US silver hake. Currently, the northern and southern populations of silver hake are considered two separate populations such that an increase in biomass in the northern population might be misinterpreted as an increase in productivity when in reality the increase in northern biomass is a result of the southern population shifting poleward [26] . Third, silver hake is both an important prey as juveniles and predator as adults in this ecosystem. With a shift in its distribution, there may be substantial changes in predator–prey dynamics and ecosystem structure. Furthermore, similar poleward shifts in distribution have been documented in many other fishes on the Northeast shelf [1] leading us to anticipate that such shifts in the GS path may be reflected in other species, altering the composition of the fish community in the Northeast US shelf region. The role of the environment has long been recognized as an important factor influencing fish production [27] . However, it has been argued that research on the effects of the environment on fish population dynamics holds little value for successfully managing living marine resources, in part, because of a lack of predictability of environmental variables, and because fishing is a more dominant driver [28] , [29] . We have shown here that the movement of a commercially important fish species tracks remote oceanographic features that are potentially predictable at decadal and multidecadal time scales through its effect on local temperature. The GS path is a large scale oceanographic feature that can be routinely measured and has the potential for predictability, because it oscillates at a decadal time scale. The decadal oscillation of the GS path and the tight correlation with silver hake distribution offer the possibility of forecasting silver hake distribution at time scales relevant to resource management (that is, 5–10 years). Finally, the established relationship between the GS path and AMOC [9] provides a way to predict the likely changes in GS path and silver hake distribution at longer time scales using sophisticated global climate models. That the spatial distribution of a commercially important fish species can be forecast by a remote oceanographic feature represents a promising advance in the way that environmental indices might be used to forecast fish distribution and abundance. Quantifying silver hake distribution and biomass Silver hake Merluccius bilinearis occurs in Northwest Atlantic offshore waters from Maryland to Labrador. Within the range of this species, three distinct populations are recognized, one population in Canada and two in the US. Division of these populations is based on discontinuous distribution between the Canadian and US stocks. In the US, identification of separate northern and southern populations ( Supplementary Fig. S2 ) was based on differential morphometric and growth characteristics in the two regions [30] . Although mixing between the populations is recognized, the northern population area includes the northern Georges Bank and Gulf of Maine area whereas the southern population area extends from southern Georges Bank to Cape Hatteras. The data to quantify silver hake spatial distribution and population size were obtained from both the spring and fall NOAA NEFSC trawl surveys, but we report only the spring time series because the timing of sampling in the spring has remained constant over time. For both surveys, only tows, in which there were no gear or duration problems from offshore trawl survey strata consistently sampled over the survey time series, were used. Correction factors were applied for vessel, gear and door changes. The NEFSC trawl survey employs a random stratified sampling design where the number of stations sampled in each strata is proportional to the area of the strata. We calculated mean-stratified BM for each population of silver hake by adjusting for the number of stations in each strata and the area of the strata using established statistical methods [31] . Mean-stratified temperature of the continental shelf was calculated in a similar manner using temperature data that were taken at the same stations where fish were collected. The biomass-weighted temperature of occurrence is termed 'catch temperature' and was calculated for both the northern and southern populations separately using equation (1): where X was the bottom temperature (°C) at each station, j was the survey year and w i was the log-transformed (log ( x +1) in kg) biomass of silver hake at each station. COM of each population was calculated in four steps. First, station latitude and longitude were converted to across-shelf and along-shelf distances from the 200-m isobath and Cape Hatteras, North Carolina. This transformation was needed because the survey follows the curvilinear shelf and straight averages of latitude and longitude can result in centres of mass on land, off the shelf and/or outside the survey area. Second, biomass-weighted mean along-shelf and across-shelf location was calculated using equation (1) where X is the parameter of interest (along-shelf location, across-shelf location). Third, biomass-weighted mean values of across-shelf and along-shelf distances were then converted back to mean latitude and mean longitude values. Fourth, distance between each centre of biomass and a fixed point (35°N latitude and 75°W longitude) was calculated to produce one metric that incorporated both along-shelf and across-shelf shifts in distribution. The fixed point roughly corresponds to Cape Hatteras, NC and is below the southernmost extent of the NEFSC trawl survey. We used the great-circle distance formula to calculate the distance from this point and called this distance the COM: where mlat is the mean latitude at the centre of abundance and mlon is the mean longitude at the centre of abundance. The value of COM was converted to kilometers by assuming the earth is spherical with a radius of 6,367 km. Quantifying silver hake recruitment We examined recruitment of silver hake using the NEFSC fall survey data, because silver hake spawn in the late spring such that the fall survey samples these juvenile fish better. The fall survey is also thought to better estimate BM of silver hake in general because more silver hake are caught in the fall versus the spring survey. Recruits (R) were defined as fish <20 cm in total length, as fish of this size would correspond to age-1 fish or younger. Spawning stock biomass (SSB) was defined as fish >20 cm. Recruitment success was evaluated using the survivor ratio (log (R/SSB+1)) in each population. Gulf Stream index Details regarding the construction of the index of the position of the north wall of the GS are given in Joyce et al . [12] and are briefly described here. Subsurface temperature data were obtained from the recently corrected temperature measurements in World Ocean Database 2009 (S. Levitus 2010, personal communication). The temperature at 200 m depth has been used as defining the region of strong flow of the GS. The 15 °C isotherm at 200 m is the isotherm at the centre of the strong horizontal gradient of the GS and demarcates the northern wall of the GS [32] , [33] . Importantly, the water mass at this depth is relatively unaffected by local diabatic processes such as seasonal warming and stratification. To develop the GS index, an Empirical Orthogonal Function analysis was used to extract the dominant mode of variability of the 200 m temperature at the mean location of the 15 °C isotherm at this depth using observations limited to the area between 55° and 75°W ( Supplementary Fig. S2 ). Quarterly or seasonal values are available for the GS index, but the spring value was used for majority of the analysis. How to cite this article: Nye, J. A. et al . Silver hake tracks changes in Northwest Atlantic circulation. Nat. Commun. 2:412 doi: 10.1038/ncomms1420 (2011).